Unexpected layers of cryptic diversity in wood whiteLeptideabutterflies Uncovering cryptic biodiversity is essential for understanding evolutionary processes and patterns of ecosystem functioning, as well as for nature conservation. As European butterflies are arguably the best-studied group of invertebrates in the world, the discovery of a cryptic species, twenty years ago, within the common wood white Leptidea sinapis was a significant event, and these butterflies have become a model to study speciation. Here we show that the so-called 'sibling' Leptidea actually consist of three species. The new species can be discriminated on the basis of either DNA or karyological data. Such an unexpected discovery challenges our current knowledge on biodiversity, exemplifying how a widespread species can remain unnoticed even within an intensely studied natural model system for speciation. Given the global biodiversity crisis [1] , [2] , [3] , cataloguing the earth's species has become a race against time. Several studies have highlighted the presence and importance of cryptic biodiversity, which might represent a substantial proportion of Earth's natural capital. An estimate of cryptic species diversity is important to better understand evolutionary processes and patterns of ecosystem functioning, while also having deep implications for nature conservation [4] , [5] . The recent increase in the number of reported cryptic species is, in large part, owing to an increasing amount of studies incorporating DNA-based techniques, including large-scale approaches such as DNA barcoding [6] , which often provide resolution beyond the boundaries of morphological information. However, documenting cryptic diversity based on DNA data alone is generally not sufficient, prompting calls for integrative morphological, ecological and molecular approaches [7] , [8] . Recent estimates on the distribution of cryptic diversity are contradictory, and are based on a thin empirical foundation [4] , [9] . In any case, it is to be expected that the highest number of yet-to-be-discovered cryptic species is concentrated in the most biodiverse and least explored regions of our planet (that is, tropical areas). In temperate regions such as Europe, it is assumed that the level of unrecognized diversity is low, not only because of lower species richness, but also because taxonomic research has been intense for many groups of organisms. Such a case is represented by butterflies, probably the best-studied group of invertebrates, which have become a flagship for insect conservation efforts in Europe [10] , [11] . The discovery of a new European species of wood white ( Leptidea sp .) at the end of the twentieth century was an important event in butterfly systematics. Leptidea sinapis (Linnaeus, 1758), a common butterfly with Palaearctic distribution was found to 'hide' a cryptic species, Leptidea reali (Reissinger, 1989) [12] , [13] . After the two species were shown to be separable based on their genitalia—but not on their wing morphology [13] —several studies revealed that L. reali is often sympatric with L. sinapis and that its distribution is almost as wide as that of L. sinapis [14] , [15] . Molecular data (allozyme markers and mitochondrial DNA) also supports the specific distinctness of L. reali [16] . Moreover, much attention has been paid to behavioural and ecological aspects of the species pair L. sinapis − L. reali , to the point that they have become a model for studying speciation in cryptic species. Such studies revealed that: a premating reproductive barrier exists (females only accept conspecific males) [17] , [18] ; the two species display only limited ecological differentiation (larval food plant preference and performance) [17] , [19] ; niche separation between the two species (forests or meadows) is not caused by fixed between-species differences [20] ; differences in phenology and voltinism are mostly the result of environmentally induced pleiotropic effects [21] ; larval diapause is determined by information from the host plant [22] ; and behavioural polyphenism has been documented in female propensity to mate [23] . In this paper, we integrate molecular (mitochondrial and nuclear DNA markers), cytological (chromosome number) and morphological data (male genitalia morphometry) to study the species pair L. sinapis − L. reali . We found an unexpected pattern showing that L. reali actually comprises two synmorphic, yet genetically and karyotypically distinct, groups, with the new cryptic entity being sister to L. sinapis + L. reali , producing what may be called nested cryptic species. Therefore, the so-called 'twin species' L. sinapis − L. reali are actually a triplet of cryptic species, a result that asks for a reconsideration of previous knowledge and exemplifies the advantages of an integrative approach when studying closely related taxa. Analysis of mitochondrial and nuclear DNA markers The Bayesian and maximum likelihood gene genealogies estimated for each of the mitochondrial (cytochrome oxidase subunit I ( COI ), NADH dehydrogenase subunit 1 ( ND1 )) and nuclear loci (internal transcribed spacer 2 ( ITS2 ), wingless ( Wg ), carbamoyl-phosphate synthetase 2/aspartate transcarbamylase/dihydroorotase ( CAD )) gave largely congruent results for the species pair L. sinapis and L. reali . Depending on their degree of variability, the markers had different resolving power, but all suggested that specimens that are morphologically attributable to L. reali (based on their genitalia) are not monophyletic. Moreover, the more variable genes COI , ND1 and ITS2 showed that L. reali formed two clades and was paraphyletic with respect to L. sinapis ( Supplementary Figs S1-S5 ). The topology of the partitioned Bayesian, maximum likelihood and maximum parsimony multi-gene trees revealed three major well-resolved clades within the L. sinapis − L. reali group ( Fig. 1 ). Whereas L. sinapis was recovered as monophyletic, specimens morphologically attributable to L. reali (based on their genitalia) formed two strongly supported clades and were paraphyletic with respect to L. sinapis . One of these clades was sister to L. sinapis and included all specimens from Spain and Italy, as well as several from southern France ( Fig. 1 ). This clade is certainly attributable to genuine L. reali , as the type locality of this species lies in the French Pyrenees [12] . The other clade of specimens with reali -like morphology consisted of samples from several countries ranging from Ireland and France in the west, to eastern Kazakhstan in the east, and was recovered as sister to L. sinapis plus genuine L. reali with good support ( Fig. 1 ). This pattern was recovered by the Bayesian coalescent-based species tree estimation as well, confirming the topological relationships of the three lineages ( Fig. 2 ). The species-tree approach is less prone to misleading results than combining data by partitions, because it incorporates uncertainty associated with gene trees (probability of unsorted ancestral polymorphism), nucleotide substitution model parameters, and the coalescent process. These results, together with the karyotypic data, strongly suggest that the non-Mediterranean clade of L. reali represents a different species. The oldest available name that we could assign to the new species is juvernica (Williams, 1946), described as a subspecies for Irish populations with reali -like morphology [14] . Therefore, in accordance with the International Code of Zoological Nomenclature, we hereafter refer to the new species as Leptidea juvernica stat. nov. 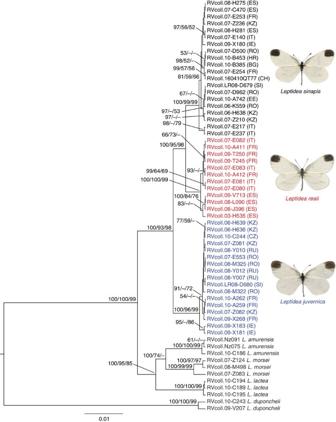Figure 1:Leptideamolecular phylogeny. Bayesian ultrametric tree based on the combined analysis ofCOI,ND1,ITS2,WgandCAD.Leptidea juvernicastat. nov. is monophyletic and sister toL. sinapis+L. reali. Bayesian posterior probabilities, maximum likelihood and maximum parsimony bootstrap values (>50%) are shown above recovered branches. IE, Ireland; ES, Spain; FR, France; IT, Italy; CH, Switzerland; SI, Slovenia; HR, Croatia; RO, Romania; BG, Bulgaria; EE, Estonia; RU, Russia; KZ, Kazakhstan. Figure 1: Leptidea molecular phylogeny. Bayesian ultrametric tree based on the combined analysis of COI , ND1 , ITS2 , Wg and CAD . Leptidea juvernica stat. nov. is monophyletic and sister to L. sinapis + L. reali . Bayesian posterior probabilities, maximum likelihood and maximum parsimony bootstrap values (>50%) are shown above recovered branches. IE, Ireland; ES, Spain; FR, France; IT, Italy; CH, Switzerland; SI, Slovenia; HR, Croatia; RO, Romania; BG, Bulgaria; EE, Estonia; RU, Russia; KZ, Kazakhstan. 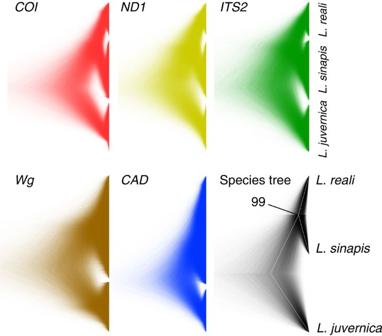Figure 2: Co-estimation of five gene trees embedded in a shared species tree. Two mitochondrial (COIandND1) and three nuclear loci (ITS2,WgandCAD) were used to estimate a species tree (in black) forL. sinapis,L. realiandL. juvernicastat. nov using *BEAST. The consensus is represented in white within the species tree and the posterior probability for theL. reali—L. sinapisclade is shown. Trees are figured with DensiTree55displaying all trees of the Markov chain Monte Carlo chain with a burn-in of 5,000 trees. Higher levels of uncertainty are represented by lower densities. Full size image Figure 2: Co-estimation of five gene trees embedded in a shared species tree. Two mitochondrial ( COI and ND1 ) and three nuclear loci ( ITS2 , Wg and CAD ) were used to estimate a species tree (in black) for L. sinapis , L. reali and L. juvernica stat. nov using *BEAST. The consensus is represented in white within the species tree and the posterior probability for the L. reali — L. sinapis clade is shown. Trees are figured with DensiTree [55] displaying all trees of the Markov chain Monte Carlo chain with a burn-in of 5,000 trees. Higher levels of uncertainty are represented by lower densities. Full size image Our sampling revealed that L. reali and L. juvernica stat. nov. display non-overlapping geographical distributions, but some populations are parapatric —at least in southeastern France, where they are separated by only 87 kilometres ( Fig. 3 , Supplementary Table S1 ). It is worth noting that we did not find any case of introgression between these two species in the parapatry zone or elsewhere. 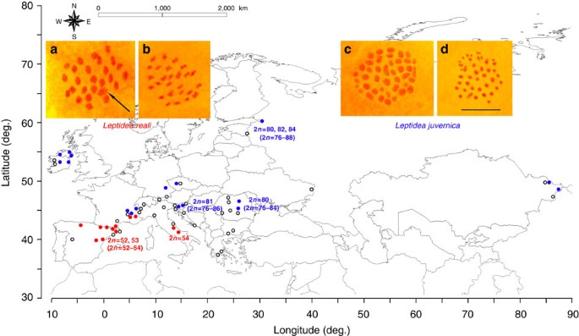Figure 3: Chromosome number results and sampling localities. Leptidea reali(red dots),L. juvernicastat. nov (blue dots) andL. sinapis(empty circles). AlthoughL. realiandL. juvernicadisplay non-overlapping distributions, they come into close contact in southeastern France and are differentiated by at least 11 fixed chromosome fusions/fissions. (a) Karyotype ofL. reali, Spain, RVcoll.03-H535: MI cell demonstrating 25 bivalents and one multivalent (most likely a trivalent, indicated by an arrow). (b)L. reali, Spain, RVcoll.07-F514: MII cell demonstrating 27 chromosomes. (c)L. juvernica, Russia, RVcoll.08-Y012: MI cell demonstrating 42 bivalents. (d)L. juvernica, Russia, RVcoll.08-Y010: MII cell demonstrating 41 chromosomes. Scale bar corresponds to 10 μm in all figures. Figure 3: Chromosome number results and sampling localities. Leptidea reali (red dots), L. juvernica stat. nov (blue dots) and L. sinapis (empty circles). Although L. reali and L. juvernica display non-overlapping distributions, they come into close contact in southeastern France and are differentiated by at least 11 fixed chromosome fusions/fissions. ( a ) Karyotype of L. reali , Spain, RVcoll.03-H535: MI cell demonstrating 25 bivalents and one multivalent (most likely a trivalent, indicated by an arrow). ( b ) L. reali , Spain, RVcoll.07-F514: MII cell demonstrating 27 chromosomes. ( c ) L. juvernica , Russia, RVcoll.08-Y012: MI cell demonstrating 42 bivalents. ( d ) L. juvernica , Russia, RVcoll.08-Y010: MII cell demonstrating 41 chromosomes. Scale bar corresponds to 10 μm in all figures. Full size image Karyotype analysis Diploid chromosome numbers 2 n =52, 2 n =53 and 2 n =54 were found in L. reali. The individuals with 2 n =52 and 2 n =54 presented 26 and 27 bivalents during first meiotic division (MI), and 26 and 27 chromosomes during second meiotic division (MII), respectively. Individuals with 2 n =53 were heterozygous for one chromosomal fusion/fission and demonstrated 25 bivalents and one trivalent in MI ( Supplementary Note 1 ). Thus, we established the chromosome number of L. reali is not fixed and ranges between 2 n =52–54. Leptidea juvernica stat. nov. displayed clearly higher chromosome numbers and, at the same time, a higher level of chromosome number variation than L. reali . We have found in mitotic cells, or have reconstructed based on meiotic cells, the following numbers: 2 n =80, 2 n =82 and 2 n =84, 2 n =ca. 81–84, 2 n =ca. 83–85. Some of the individuals studied were chromosomal heterozygotes displaying up to six multivalents in metaphase I of meiosis ( Supplementary Note 1 ). Given the karyotypes observed in MI and MII cells and taking into account all possible combinations of gametes, we concluded that chromosome numbers ranging from 2 n =76 to 2 n =88 are expected to be found in L. juvernica stat. nov. Our results show that L. reali and L. juvernica stat. nov. are differentiated by at least 11 chromosomal fusions/fissions. Morphological analysis The Shapiro-Wilk test supported normal distributions for the five measured variables (phallus length (PL), saccus length (SL), vinculum width (VW), genital capsule length and uncus length (UL)) ( P >0.05). For the discriminant analysis, the variables included in the prediction equation with the stepwise method and using Wilks' Lambda were PL, VW and SL. The first two canonical discriminant functions explained 100% of the variance and were used in the analysis. The first function alone accounted for 99.4% of the variance displaying a strong canonical correlation of 0.951 and a highly significant Wilks' Lambda (0.091, P <0.001). The second function explained 0.6% of the variance, displayed a canonical correlation of 0.227 and had a significant Wilks' Lambda (0.949, P =0.032). The structure matrix that was obtained ( Supplementary Table S2 ) showed the canonical weight of each variable which is an indicator of its discriminatory power. All specimens attributed to L. sinapis in the molecular analysis were correctly classified by the discriminant analysis, supporting previous results indicating that male genitalia allow for the separation of L. sinapis and L. reali sensu lato . On the other hand, classification was much less accurate for L. reali and L. juvernica stat. nov. (61.5% for L. reali and 62.5% for L. juvernica with 53.8% and 58.3%, respectively, after cross validation) ( Fig. 4 , Supplementary Table S3 ), indicating that they cannot be reliably identified based on the parameters involved. To further test these results, another discriminant analysis was run including only L. reali and L. juvernica stat. nov. Two variables were introduced in the prediction equation: SL and genital capsule length (GL). The first function explained 100% of the variance and was used in the analysis. This function displayed a moderate canonical correlation of 0.357 and a significant Wilks' Lambda of 0.873 ( P =0.003). Classification results were similar to the previous analysis, with 56.4% of L. reali and 64.6% of L. juvernica stat. nov. correctly identified (53.8% and 62.5%, respectively, after cross-validation). This confirmed that, although there seemed to be a slight tendency of larger genitalia for L. reali specimens ( Fig. 4 ), identification was unreliable based on male genitalia. 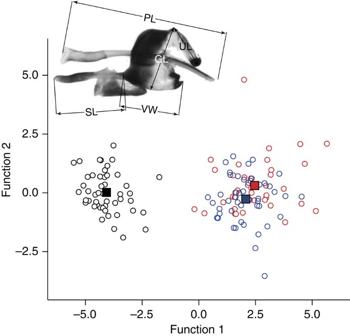Figure 4: Discriminant analysis based on male genitalia morphometry. L. sinapis(black) is identifiable based on male genitalia, but there is broad overlap betweenL. reali(red) andL. juvernicastat. nov (blue). Circles represent individuals and squares represent centroids for each species. Elements of the male genitalia measured were PL, SL, VW, GL and UL. The discriminant variables were PL and SL for function 1 and SL and VW for function 2. The upper left corner image indicates the variables measured forLeptideamale genitalia. Figure 4: Discriminant analysis based on male genitalia morphometry. L. sinapis (black) is identifiable based on male genitalia, but there is broad overlap between L. reali (red) and L. juvernica stat. nov (blue). Circles represent individuals and squares represent centroids for each species. Elements of the male genitalia measured were PL, SL, VW, GL and UL. The discriminant variables were PL and SL for function 1 and SL and VW for function 2. The upper left corner image indicates the variables measured for Leptidea male genitalia. Full size image Female genitalia of a few specimens corresponding to L. reali and L. juvernica stat. nov. were also examined. Although our sample was too small to permit statistical analyses, we did not notice any apparent difference in the length of the ductus bursae, the most useful character to discriminate females of L. sinapis from L. reali [13] , [24] . This study presents strong evidence for the existence of a previously unnoticed, widespread species of Leptidea . This is clearly supported by our combined molecular phylogeny based on two mitochondrial and three nuclear markers, as well as by the coalescent-based species tree reconstruction, which showed that the new species L. juvernica stat. nov. is sister to the species pair L. sinapis and L. reali . No topological discordance in the relationships among the three species was detected in the single-gene trees ( Fig. 2 ), except for CAD and Wg , which mixed specimens of L. sinapis and L. reali . The slower mutation rate and/or coalescent process of these two nuclear markers is most probably the cause, but it is worth noting that they recovered the new species as a different entity. When combining the three nuclear loci, the monophyly of all species was strongly supported ( Supplementary Fig. S6 ). Our conclusions based on molecular data were also supported by karyotype analyses, which revealed different chromosome numbers between L. reali (2 n =52–54) and L. juvernica stat. nov. (2 n =80–84). Although the chromosome number is not fixed in these species, intraspecific variation is limited and the interspecific gap is pronounced (at least 11 chromosomal rearrangements). It is relevant that karyotype characteristics (chromosome numbers and level of chromosome number variability) are nearly identical in geographically distant populations within each species, whereas L. reali from Italy and L. juvernica stat. nov. from Slovenia are drastically different, despite geographical proximity. Mating between species with different karyotypes is known to produce hybrids that are heterozygous for chromosomal rearrangements fixed between parental species. These hybrids typically have reduced fertility due to partial missegregation of homologous chromosomes during the MI [25] . Although different kinds of chromosomal rearrangements have various effects on the fertility of heterozygous hybrids [26] , hybrid fertility is generally negatively correlated with the extent of karyotypic divergence between parental taxa [27] , [28] , and multiple chromosome fusion/fissions, such as those we detected in L. reali and L. juvernica stat. nov., can strongly contribute to postzygotic reproductive isolation. Although we have no direct data on the degree of postzygotic isolation, the chromosomal differentiation between L. reali and L. juvernica stat. nov. is high and can be considered as additional independent evidence that there are two distinct species. Morphometry results showed that specimens of L. reali and L. juvernica cannot be reliably distinguished, whereas L. sinapis was clearly differentiated based on genitalic measurements. Wing and preimaginal stage morphology did not appear to be useful for identification either, as already shown by several studies comparing L. sinapis and L. reali sensu lato [13] . Therefore, L. reali and L. juvernica stat. nov. seem to represent the plesiomorphic state and to have remained in morphological stasis, wheras L. sinapis evolved genitalic differences. The fact that the new cryptic species reported here is apparently fully synmorphic to L. reali explains why it remained unnoticed for such a long time despite intensive research. We propose the common name 'cryptic wood white' for L. juvernica stat. nov. The relationships between the three studied species suggest that the common ancestor of the triplet of species (ancestor A) ( Fig. 5a,b ) probably originated in central or western Asia and subsequently spread over western Europe. The hypothesis of an eastern origin is also supported by the exclusively eastern distribution of the closest relatives ( L. amurensis , L. morsei and L. lactea ) to the triplet of cryptic species ( Fig. 1 ). About 270,000 years ago ( Supplementary Table S4 ), probably in southwestern Europe, ancestor A speciated producing the common ancestor of L. sinapis and L. reali (ancestor B), and the L. juvernica stat. nov. lineage that established across temperate Europe and Asia ( Fig. 5c ). About 120,000 years ago, ancestor B diverged into L. sinapis and L. reali ( Fig. 5d ). Later on (ca. 27,000 years ago), L. sinapis expanded north and east into the territory of L. juvernica stat. nov. ( Fig. 5e ). On the basis of our sampling, L. reali and L. juvernica stat. nov. are most likely parapatric, with L. reali confined to southwestern Europe and L. juvernica stat. nov. spread across temperate Europe and Asia. This provides a totally new view on L. reali which is actually a west Mediterranean species and not a widely distributed taxon as concluded before. Our sampling suggests a potential contact zone in southeastern France, where populations of the two species are separated by less than 90 kilometres ( Fig. 3 ). 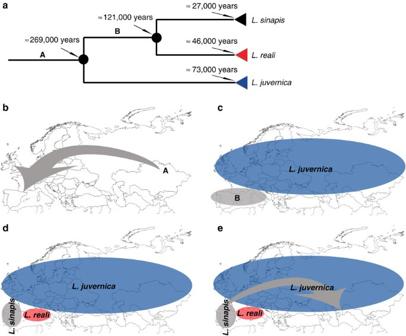Figure 5: Phylogenetic relationships and proposed speciation scenario. (a)L. juvernicastat. nov is sister toL. sinapis+L. reali. Age estimations are indicated for each node. (b) The common ancestor of the whole group (ancestor A) probably originated in central or western Asia and subsequently colonized western Europe. (c) Ancestor A split intoL. juvernicain temperate Europe and Asia and the common ancestor ofL. sinapisandL. reali(ancestor B) in southwestern Europe (d) Ancestor B speciated intoL. sinapisandL. reali. (e) Subsequently,L. sinapisrapidly spread north and east into the territory ofL. juvernica. Figure 5: Phylogenetic relationships and proposed speciation scenario. ( a ) L. juvernica stat. nov is sister to L. sinapis + L. reali . Age estimations are indicated for each node. ( b ) The common ancestor of the whole group (ancestor A) probably originated in central or western Asia and subsequently colonized western Europe. ( c ) Ancestor A split into L. juvernica in temperate Europe and Asia and the common ancestor of L. sinapis and L. reali (ancestor B) in southwestern Europe ( d ) Ancestor B speciated into L. sinapis and L. reali . ( e ) Subsequently, L. sinapis rapidly spread north and east into the territory of L. juvernica . Full size image To know the causes behind the apparent inability of L. reali and L. juvernica stat. nov. to coexist will require further studies. It has been shown that, besides differences in the genitalia, behavioural aspects related to mate choice maintain reproductive isolation between L. sinapis and L. reali sensu lato [17] , [18] . Previous data on the biology and ecology of L. reali sensu lato , as well as our view of the speciation processes undergone by Leptidea , need to be extensively revised in light of these results [17] , [18] , [19] , [20] , [21] , [22] , [23] , [29] . Our observations revealed that both L. reali and L. juvernica stat. nov. can use Lathyrus pratensis as a larval food plant (oviposition observed in Spain for L. reali and in Romania for L. juvernica stat. nov. and adults obtained from these eggs by rearing in the laboratory). It is thus to be expected that ecological differentiation between the two species is minimal. In this study, we show that assessing cryptic diversity is a challenging task even in well-studied groups of organisms. What has been formerly called the cryptic species pair, L. sinapis − L. reali comprises a triplet of species, and new research is needed to clarify their distribution, ecology and conservation status. Our findings exemplify that cryptic biodiversity may consist of finely nested layers and highlight the importance of using an array of techniques when dealing with closely related species. Specimen sequencing The mitochondrial marker COI was sequenced in 166 specimens, the mitochondrial ND1 in 85 specimens, the nuclear ITS2 in 91 specimens, the nuclear wingless ( Wg ) in 67 specimens and the nuclear CAD in 43 specimens. Thirteen GenBank COI sequences of L. sinapis from Spain [30] , France [31] , Slovenia [32] , Greece [21] and Kazakhstan [33] , seven sequences of L. juvernica stat. nov. from Slovenia [32] , three sequences of L. amurensis [33] from Russia and two sequences of L. morsei [33] from Kazakhstan were also added to the dataset. Additionally, one sequence of L. sinapis from Austria and three sequences of L. juvernica stat. nov. from Germany were included from the publicly available project 'Fauna Bavarica—Lepidopera Rhopalocera' included in the Barcode of Life Data System at www.barcodinglife.org . Four ND1 Leptidea GenBank sequences (two L. reali and two L. sinapis ) [16] were also added to the dataset. All novel sequences obtained in this study have been deposited to GenBank under accession codes JF512569 to JF513007 (for details see Supplementary Table S1 ). Total genomic DNA was extracted using Chelex 100 resin, 100–200 mesh, sodium form (Bio-rad), under the following protocol: one leg was removed and introduced into 100 μl of Chelex 10% and 5 μl of Proteinase K (20 mg ml −1 ) were added. The samples were incubated overnight at 55 °C and were subsequently incubated at 100 °C for 15 min. Afterwards they were centrifuged for 10 s at 3,000 r.p.m. The primers used were: for COI (676 bp) LCO 1490 (5′-GGTCAACAAATCATAAAGATATTGG-3′) [34] and Nancy (5′-CCCGGTAAAATTAAAATATAAACTTC-3′) [35] , or (658 bp) LepF1 (5′-ATTCAACCAATCATAAAGATATTGG-3) and LepR1 (5′-TAAACTTCTGGATGTCCAAAAAATCA-3′) [36] ; for ND1 (790–794 bp) 5′- CTGTTCGATCATTAAAATCTTAC-3′ (forward) [37] and 5′-ATCAAAAGGAGCTCGATTAGTTTC-3′ (reverse) [38] ; for ITS2 (684 bp) ITS3 (5′-GCATCGATGAAGAACGCAGC-3′) and ITS4 (5′-TCCTCCGCTTATTGATATGC-3′) [39] ; for Wg (403 bp) Wg1 (5′-GARTGYAARTGYCAYGGYATGTCTGG-3′) and Wg2 (5′-ACTICGCRCACCARTGGAATGTRCA-3′) [40] ; for CAD (571 bp) CADFa (5′-GDATGGTYGATGAAAATGTTAA-3′) and CADRa (5′-CTCATRTCGTAATCYGTRCT-3′). Double-stranded DNA was amplified in 25 μl volume reactions: 13.22 μl ultra pure (HPLC quality) water, 2.5 μl 10× buffer, 4.5 μl 25 mM MgCl 2 , 0.25 μl 100 mM dNTP, 1.2 μl of each primer (10 mM), 0.13 μl Taq DNA Gold Polymerase (Qiagen) and 2 μl of extracted DNA. The typical thermal cycling profile for COI was 95 °C for 60 s, 44 °C for 60 s and 72 °C for 90 s, for 40 cycles. The annealing temperature varied according to marker: 48 for ND1 , 47 for ITS2 , 51 for Wg , and 48 for CAD . PCR products were purified and sequenced by Macrogen Inc. All the samples are stored in the Institut de Biologia Evolutiva collection in Barcelona, Spain, and are available upon request. Phylogenetic analyses and species tree estimation COI , ND1 , ITS2 , Wg and CAD sequences were edited and aligned using Geneious Pro 4.7.5 [41] . These resulted in five alignments of 676 bp and 195 specimens for COI , 794 bp and 89 specimens for ND1 , 715 bp and 91 specimens for ITS2 , 403 bp and 67 specimens for Wg , and 571 bp and 43 specimens for CAD . For COI , duplicate haplotypes (excluding outgroups) were removed using TCS 1.21 [42] . Individual Bayesian and ML phylogenetic trees were inferred using COI , ND1 , ITS2 , Wg , and CAD with BEAST 1.6.0 [43] and GARLI 1.0 [44] . Relationships based on the combined dataset were estimated using partitioned Bayesian and ML analyses using BEAST 1.6.0 and GARLI-PART v. 0.97 [44] with substitution models by markers according to the suggestions of jModeltest 0.1 [45] . The models employed for the partitioned ML analysis were TPMuf+I+G for COI , HKY+I for CAD and ND1 , TVM for ITS2 and TPM2 for Wg . For the partitioned BI, GTR+I+G was used for COI , HKY+I for CAD and ND1 , GTR for ITS2 and HKY for Wg . Branch support was assessed by 100 bootstrap replicates for maximum likelihood, and Markov chain Monte Carlo convergence was checked after two independent runs of 10 million generations each (with a pre-run burn in of 100,000 generations) for Bayesian inference. A multilocus coalescent-based Bayesian species tree was estimated with *BEAST [46] . L. sinapis , L. reali and L. juvernica stat. nov. specimens were defined as three taxonomic units in accordance with clades previously inferred by single-gene and five-loci combined trees. A relaxed clock with uncorrelated lognormal distribution [47] and a Yule speciation process as tree prior were used. The length of the Markov chain Monte Carlo chain was set at 50 million generations sampling every 1,000 runs with a burn-in set to the first 500,000 generations. A maximum parsimony tree based on the five markers combined was inferred with MEGA4 [48] and branch supports were assessed by 100 bootstrap replicates. Dating divergence events Node ages were inferred with BEAST 1.6.0 [43] using the COI haplotype dataset under a coalescent model with constant population size. We calibrated the phylogeny at two selected nodes: the L. sinapis common ancestor node as an example of a very recent clade supposedly under a coalescent process, and the root of the tree as a clearly coalesced node. For the age of the root node, we used a normally distributed prior ranging between 2.2 and 4 MYA based on slow and fast published invertebrate mitochondrial rates of 1.3 and 2.3% uncorrected pairwise distance per million years [49] , [50] . The prior range assumed for the common ancestor of L. sinapis was a normal distribution between 8,500–31,000 years, as previously inferred [51] . The dataset was analysed using the GTR+I+G model and applying an uncorrelated lognormal relaxed molecular clock [47] along the branches. Base frequencies were estimated, six gamma rate categories were selected and a randomly generated initial tree was used. Parameters were estimated using two independent runs of 10 million generations each (with a pre-run burn in of 100,000 generations) to ensure convergence, and were checked with the program Tracer v1.5. Karyotype analyses Gonads were stored in Carnoy fixative (ethanol and glacial acetic acid, 3:1) for 2–6 months at 4 °C and then stained with 2% acetic orcein for 30 days at 20 °C. Cytogenetic analysis was conducted using a two-phase method of chromosome analysis [52] . In our study, we have counted the diploid chromosome numbers (2n) in mitotic spermatogonial cells and the haploid chromosome numbers (n) in metaphase II of male meiosis. We also counted the number of chromosomal elements (n) (bivalents+multivalents) in metaphase I of male meiosis. In the last case, the number of chromosomal elements was equal to the haploid number (n), if all the elements were represented by bivalents, or less if some elements were represented by multivalents. To distinguish between bivalents and multivalents, we used a special method [53] . Briefly, by varying the pressure on the coverslip, we were able to manipulate chromosomes, for example, change their position and orientation in intact (not squashed) spermatocyte cells, and consequently to analyse the structure of the bivalents and multivalents. In total, preparations from 68 males were analysed. As cell divisions are extremely rare in Leptidea during imago stage [54] , metaphase plates were observed in only 14 individuals ( Supplementary Table S1 ). These individuals have also been used for morphological and molecular analysis. Genitalia preparation and morphometrics Male genitalia were prepared according to the following protocol: maceration for 15 min at 95 °C in 10% potassium hydroxide, dissection and cleaning under a stereomicroscope and storage in tubes with glycerine. Genitalia were photographed in a thin layer of distilled water (without being pressed under a cover slip) under a Carl Zeiss Stemi 2000-C stereomicroscope equipped with a DeltaPix Invenio 3S digital camera. Measurements were performed based on the digital photographs by using AxioVision software. A total of 39 specimens of L. reali , 48 of L. juvernica stat. nov. and 48 of L. sinapis were included in the morphometrical analyses ( Supplementary Table S5 ). Five elements of the male genitalia were measured: PL, SL, VW, GL (measured from the ventral edge of the vinculum to the uncus apex) and UL. The first three elements combined were reported to be the best to discriminate between L. sinapis and L. reali [13] , [16] , [24] . Statistical analyses were carried out using the software SPSS 14.0 for Windows. The first batch of analyses was run by including three groups: Leptidea reali , L. juvernica stat. nov. and L. sinapis . Subsequently the analyses were repeated including only L. reali and L. juvernica stat. nov. A Shapiro-Wilk normality test was employed. Subsequently, a discriminant analysis was performed by employing the stepwise method. In order to test the obtained classification, a cross validation was carried out ('leave-one-out' method). Accession Codes: All novel sequences obtained in this study have been deposited to GenBank under accession codes JF512569 to JF513007 . How to cite this article: Dincă, V. et al . Unexpected layers of cryptic diversity in wood white Leptidea butterflies. Nat. Commun. 2:324 doi: 10.1038/ncomms1329 (2011).